A steep-slope transistor based on abrupt electronic phase transition Collective interactions in functional materials can enable novel macroscopic properties like insulator-to-metal transitions. While implementing such materials into field-effect-transistor technology can potentially augment current state-of-the-art devices by providing unique routes to overcome their conventional limits, attempts to harness the insulator-to-metal transition for high-performance transistors have experienced little success. Here, we demonstrate a pathway for harnessing the abrupt resistivity transformation across the insulator-to-metal transition in vanadium dioxide (VO 2 ), to design a hybrid-phase-transition field-effect transistor that exhibits gate controlled steep (‘sub- kT/q ’) and reversible switching at room temperature. The transistor design, wherein VO 2 is implemented in series with the field-effect transistor’s source rather than into the channel, exploits negative differential resistance induced across the VO 2 to create an internal amplifier that facilitates enhanced performance over a conventional field-effect transistor. Our approach enables low-voltage complementary n-type and p-type transistor operation as demonstrated here, and is applicable to other insulator-to-metal transition materials, offering tantalizing possibilities for energy-efficient logic and memory applications. Metal-oxide-semiconductor field-effect transistors (MOSFETs) have been the workhorse of digital computation. In a conventional MOSFET ( Fig. 1a ), a change in the drain-to-source current ( I DS ) can be induced by the application of a transverse electric field across the gate dielectric by means of the third gate terminal. This field lowers the potential energy barrier separating the source and the channel, exponentially increasing the number of carriers traversing the channel. At room temperature, a minimum change of 60 mV in the gate bias ( V GS ) is required to effectuate a decade change in I DS , setting up the so-called ‘60 mV per decade’ limit, also known as the ‘Boltzmann limit’ ( Fig. 1a ). Stemming from the statistical distribution of free and independent carriers in conventional semiconductors and determined by the thermal voltage kT / q ( k : Boltzmann constant; T : temperature; q : electron charge), this fundamental limit restricts transistor performance, particularly at low-operating voltages [1] , [2] , [3] , [4] , and has motivated the exploration of FETs that harness collective carrier responses [5] , [6] , [7] , [8] , [9] , [10] , [11] , [12] , [13] . Such collective behaviour—wherein a small external perturbation can trigger an aggregated change in the ground state of the system—can produce internal amplification; and provide a pathway to overcome the Boltzmann limit to enable FET’s with sub- kT / q ( kT / ηq ; η >1) switching slope and superior performance at low voltages. Particularly, in insulator-to-metal transition (IMT) materials [14] that exhibit strong correlation, like VO 2 (refs 15 , 16 , 17 , 18 ), the collective response to external perturbation (temperature [19] , [20] , pressure [21] , [22] and electrical stimulus [23] , [24] , [25] , [26] , [27] , [28] ) can be the ‘melting’ of carriers, marking an electronic phase transformation where the electrons localized at atomic sites change to an itinerant state ( Fig. 1b ). This phase transformation amplifies the free-carrier concentration [29] ; and in the case of VO 2 , manifests itself as a sharp change in resistivity up to five orders in magnitude [30] at ∼ 340 K. However, attempts to realize IMT-based three-terminal transistor devices with a solid-state gate dielectric to induce the phase transition directly in the channel material have experienced only limited success [23] , [31] , [32] , [33] . Further, the alternate approach of using an ionic liquid as the gate dielectric, which is the focus of current research [34] , [35] , [36] , [37] , [38] , [39] , is typically slow [40] , [41] , [42] and susceptible to electrochemical effects [43] . These constraints have restricted the utilization of this collective phenomenon in FETs for advanced high-performance electronic applications. 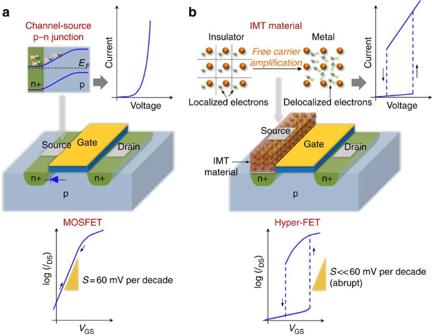Figure 1: Schematic device design of hyper-FET and working principle. (a) Conventional MOSFET and its transfer characteristics (channel currentIDSversus gate biasVGS) for a fixed drain-to-source voltageVDS. The channel-source p–n junction, modulated by the gate terminal, controls the injection of carriers into the channel limiting the switching slope (S) of the MOSFET to 60 mV per decade (Boltzmann limit). (b) Proposed hyper-FET in which an insulator-to-metal transition (IMT) material that shows electrically induced abrupt resistivity switching is electrically integrated in series with the source of a conventional MOSFET. For a givenVDS, the gate-terminal voltageVGSmodifies the current flowing through the MOSFET and the IMT material in series, triggering an abrupt phase transition. The associated delocalization of localized carriers (free-carrier amplification) across the IMT results in an abrupt decrease in the resistance of the source, enhancing the switching slope characteristics beyond the intrinsic limits of a conventional p–n junction. Figure 1: Schematic device design of hyper-FET and working principle. ( a ) Conventional MOSFET and its transfer characteristics (channel current I DS versus gate bias V GS ) for a fixed drain-to-source voltage V DS . The channel-source p–n junction, modulated by the gate terminal, controls the injection of carriers into the channel limiting the switching slope ( S ) of the MOSFET to 60 mV per decade (Boltzmann limit). ( b ) Proposed hyper-FET in which an insulator-to-metal transition (IMT) material that shows electrically induced abrupt resistivity switching is electrically integrated in series with the source of a conventional MOSFET. For a given V DS , the gate-terminal voltage V GS modifies the current flowing through the MOSFET and the IMT material in series, triggering an abrupt phase transition. The associated delocalization of localized carriers (free-carrier amplification) across the IMT results in an abrupt decrease in the resistance of the source, enhancing the switching slope characteristics beyond the intrinsic limits of a conventional p–n junction. Full size image Here, we explore a novel transistor architecture that harnesses the abrupt free-carrier amplification across the phase transition in VO 2 using a conventional MOSFET. By electrically coupling the VO 2 in series with the source of a conventional MOSFET ( Fig. 1b ), we design a hybrid-phase-transition-FET (hyper-FET) wherein, for a given drain-to-source voltage ( V DS ), the gate bias V GS modifies the current I DS flowing through the MOSFET channel and the VO 2 in series, triggering an abrupt phase transformation in VO 2 . The proposed hyper-FET not only exhibits steep-slope characteristics but also circumvents the need for a direct field-induced phase transition in VO 2 with a solid-state gate dielectric. Further, the abrupt resistivity switching of VO 2 in the hyper-FET configuration, which is the origin of the steep-slope characteristics, induces a negative differential resistance (NDR) across VO 2 that results in internal voltage amplification which consequently enhances the hyper-FET’s performance beyond that of a conventional MOSFET. 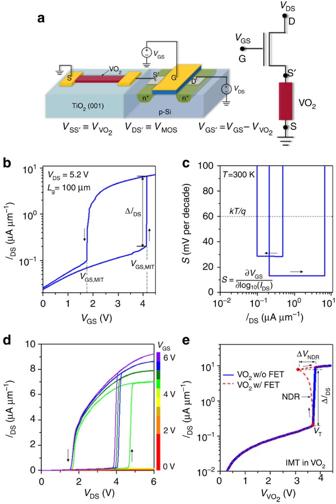Figure 2: Experimental demonstration of a VO2-based hyper-FET. (a) Schematic of a hyper-FET consisting of a two-terminal VO2device (=4 μm;=2 μm) in series with the channel of a conventional Si n-MOSFET (Lg=100 μm;W=100 μm). VVO2is the voltage across the VO2device andVGS′is the effective gate-to-source voltage across the MOSFET. (b)IDS–VGStransfer characteristics of the hyper-FET exhibiting abrupt and reversible modulation of the channel currentIDSas a function of the gate-source voltageVGS. The abrupt turn-ON and turn-OFF of the hyper-FET corresponds to the IMT and MIT in VO2, respectively. (c) Switching slope (S) as a function ofIDSrevealing the steep-slope characteristics (S<60 mV per decade) of the hyper-FET during the forward and reverse gate bias sweep. (d) Output characteristics (IDS–VDS) of the hyper-FET with excellent current saturation. (e) Current versus voltage characteristics of the VO2device with (red) and without (blue) the MOSFET in series, illustrating the electrically triggered abrupt IMT. The channel resistance of the MOSFET acts as a series resistor, modifying the current–voltage dynamics through a feedback and inducing a negative differential resistance NDR (red) across the phase transition in VO2. The NDR reduces the voltage across the VO2by ΔVNDR. The current has been normalized to the width of the Si n-MOSFET to show that the abrupt IMT in VO2triggers the abrupt turn-ON of the hyper-FET shown inb. Experimental demonstration and operation principle Figure 2a illustrates the schematic of an experimental hyper-FET consisting of a two-terminal VO 2 device in series with the channel of a conventional Si n-MOSFET (individual device characteristics are shown in Supplementary Fig. 1 and discussed in Supplementary Note 1 ). All measurements in this work are performed at room temperature ( T =300 K). The modulation in the transfer characteristics ( I DS – V GS ) of the hyper-FET is shown in Fig. 2b . Initially, at V GS =0 V (MOSFET in OFF-state), VO 2 is in the high-resistivity insulating state. In this series combination, V DS is divided between the MOSFET channel and the insulating VO 2 in proportion to their respective resistances; and the current I DS through the channel and VO 2 is insufficient to induce an IMT. As V GS increases, the MOSFET-channel resistance decreases until I DS reaches a critical current threshold, I IMT . This triggers an abrupt IMT with the VO 2 transforming into the low-resistivity metallic state that consequently leads to an abrupt increase in I DS (turn-ON). Similarly, as V GS reduces, the MOSFET-channel resistance increases until I DS drops to a critical threshold value, I MIT , and the VO 2 transforms back to the high-resistivity insulating state accompanied by an abrupt reduction in I DS (turn-OFF). The difference between the critical threshold values ( I MIT > I IMT ; corresponding to V GS,IMT , V GS,MIT , respectively) results in hysteresis (= V GS,IMT − V GS,MIT ) ( Fig. 2b ). Figure 2: Experimental demonstration of a VO 2 -based hyper-FET. ( a ) Schematic of a hyper-FET consisting of a two-terminal VO 2 device ( =4 μm; =2 μm) in series with the channel of a conventional Si n-MOSFET ( L g =100 μm; W =100 μm). V VO 2 is the voltage across the VO 2 device and V GS′ is the effective gate-to-source voltage across the MOSFET. ( b ) I DS – V GS transfer characteristics of the hyper-FET exhibiting abrupt and reversible modulation of the channel current I DS as a function of the gate-source voltage V GS . The abrupt turn-ON and turn-OFF of the hyper-FET corresponds to the IMT and MIT in VO 2 , respectively. ( c ) Switching slope ( S ) as a function of I DS revealing the steep-slope characteristics ( S <60 mV per decade) of the hyper-FET during the forward and reverse gate bias sweep. ( d ) Output characteristics ( I DS – V DS ) of the hyper-FET with excellent current saturation. ( e ) Current versus voltage characteristics of the VO 2 device with (red) and without (blue) the MOSFET in series, illustrating the electrically triggered abrupt IMT. The channel resistance of the MOSFET acts as a series resistor, modifying the current–voltage dynamics through a feedback and inducing a negative differential resistance NDR (red) across the phase transition in VO 2 . The NDR reduces the voltage across the VO 2 by Δ V NDR . The current has been normalized to the width of the Si n-MOSFET to show that the abrupt IMT in VO 2 triggers the abrupt turn-ON of the hyper-FET shown in b . Full size image Analysing the switching slope , shown in Fig. 2c , it is evident that the abrupt change in current associated with the IMT/MIT in VO 2 results in steep-slope ( S <60 mV per decade) characteristics, both during the forward and the reverse V GS sweep. We emphasize that the current change Δ I DS is abrupt and the extracted value of S is limited by the voltage resolution (1 mV). The corresponding output characteristics ( I DS – V DS ) of the hyper-FET ( Fig. 2d ) show excellent I DS saturation behaviour, which is paramount for small signal amplification. This is in contrast to the traditional IMT-based transistor design where the IMT occurs in the channel material [23] . Such a transistor is unlikely to demonstrate current saturation since the design envisages the IMT channel to have a metallic character in the transistor’s ON-state which fundamentally cannot sustain a drain side depletion region. Internal amplification in the hyper-FET To elucidate the internal amplification, we analyze the current–voltage dynamics across VO 2 in the hyper-FET configuration ( Fig. 2e ). In this series combination, the abrupt IMT results in an NDR across the VO 2 . Such an NDR is induced because when the VO 2 resistance decreases abruptly, it results in (a) an increase in I DS (Δ I DS ) which flows through the VO 2 device and the MOSFET channel in series; (b) a reduction in the voltage across the VO 2 device (−Δ V NDR ) (see Supplementary Fig. 2 and Supplementary Note 2 for discussion on the NDR in VO 2 ). The effective gate-to-source voltage across the MOSFET ( V GS′ ; S′: internal node in Fig. 2a ) when VO 2 is in the insulating state (hyper-FET OFF-state) is V GS′ = V GS − . It can be observed that the voltage across the insulating VO 2 results in an additional voltage drop (=− ) in the effective gate-to-source voltage V GS′ . Across the IMT in VO 2 which induces the NDR, this voltage drop (=− ) reduces by Δ V NDR (therefore increasing V GS′ by Δ V NDR ; Fig. 2a ). Thus, the additional voltage drop (=− ) in V GS′ when VO 2 is in the insulating state results in a drastic reduction in the OFF-state current ( I DS,OFF ) of the hyper-FET in comparison to the stand-alone MOSFET, whereas the reduction in ON-state current ( I DS,ON ) is much less significant since the voltage drop across the metallic VO 2 is small; this results in an overall enhanced current change that is, a higher I DS,ON / I DS,OFF ratio (see Supplementary Fig. 3 and Supplementary Note 3 for additional details and simulations). We model the MOSFET with VO 2 combination as an equivalent common-source transistor circuit ( Fig. 2a ) where: Here, g m is the transconductance of the stand-alone MOSFET. Across the IMT, the VO 2 exhibits an NDR ( =−Δ V NDR /Δ I DS ), and therefore equation (1) evolves to: where Equation (2) indicates that in a particular gate-voltage window, the amplified differential transconductance ( βg m ; β >1) of the hyper-FET facilitates a larger change in current compared with the stand-alone MOSFET. The VO 2 , therefore, sets up an internal amplifier ( β >1) in the hyper-FET, and the transconductance enhancement ( βg m ) is directly related to the free-carrier amplification across the phase transition. We note that although the hyper-FET has reduced transconductance before and after the IMT (that is, VO 2 in the stable insulating/metallic state), the abrupt free-carrier amplification across the IMT overcompensates this reduction and enables an amplified current change. To evaluate the improved performance of the hyper-FET, particularly for digital-logic applications, we match the OFF-state current I DS,OFF of the hyper-FET and the stand-alone MOSFET and analyze the increase in ON-state current I DS,ON over the operating gate-voltage window, as shown further. Low-voltage n-type and p-type hyper-FET operation Next, we focus on the MOSFET component of the hyper-FET. The gate-bias triggers the phase transition in VO 2 by enabling the MOSFET to source the corresponding critical currents. Therefore, using a scaled transistor can enable low-voltage hyper-FET operation since the transistor can now source the same currents at low V GS and V DS . This motivates the integration of scaled, high- g m -advanced transistor architectures like FinFETs fabricated on channel materials having mobilities higher than that of silicon to design a low-voltage hyper-FET ( Figs 3 and 4 ). 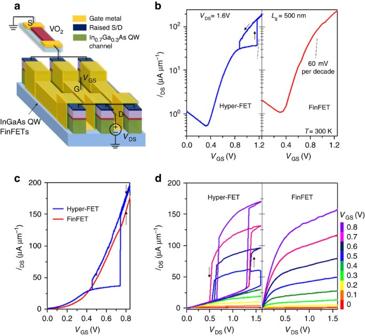Figure 3: Experimental demonstration a low-voltage hyper-FET using next generation FinFET technology beyond Si. (a) Schematic of the n-hyper-FET consisting of a series combination of a scaled VO2(=200 nm) and a multi-channel (=3 fins) In0.7Ga0.3As quantum-well FinFET (Lg=500 nm). (b) Transfer characteristics (IDS–VGS) of the hyper-FET and the stand-alone FinFET. (c) The positive feedback provided by the VO2enables the hyper-FET to exhibit a∼20 % higher ON-state current (IDS,ON) compared with the stand-alone n-FinFET over a gate-voltage window of 0.8 V at matched OFF-state current. (d) Output characteristics (IDS–VDS) of the n-hyper-FET and the conventional FinFET. Figure 3: Experimental demonstration a low-voltage hyper-FET using next generation FinFET technology beyond Si. ( a ) Schematic of the n-hyper-FET consisting of a series combination of a scaled VO 2 ( =200 nm) and a multi-channel (=3 fins) In 0.7 Ga 0.3 As quantum-well FinFET ( L g =500 nm). ( b ) Transfer characteristics ( I DS – V GS ) of the hyper-FET and the stand-alone FinFET. ( c ) The positive feedback provided by the VO 2 enables the hyper-FET to exhibit a ∼ 20 % higher ON-state current ( I DS,ON ) compared with the stand-alone n-FinFET over a gate-voltage window of 0.8 V at matched OFF-state current. ( d ) Output characteristics ( I DS – V DS ) of the n-hyper-FET and the conventional FinFET. 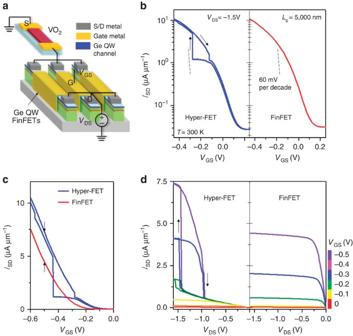Figure 4: Experimental demonstration of a low-voltage p-type hyper-FET. (a) Schematic of the p-hyper-FET consisting of a series combination of scaled VO2(=200 nm) and multi-channel (=200 fins) p-type Ge quantum-well FinFET (Lg=5,000 nm). (b) Transfer characteristics (ISD–VGS) of the hyper-FET and the FinFET (stand-alone). (c) The p-hyper-FET shows a∼60 % higher ON-state current (ISD,ON) in comparison to the stand-alone FinFET over a gate-voltage window of −0.5 V at matched OFF-state current. (d) Output characteristics (ISD–VDS) of the p-hyper-FET and the conventional FinFET. Full size image Figure 4: Experimental demonstration of a low-voltage p-type hyper-FET. ( a ) Schematic of the p-hyper-FET consisting of a series combination of scaled VO 2 ( =200 nm) and multi-channel (=200 fins) p-type Ge quantum-well FinFET ( L g =5,000 nm). ( b ) Transfer characteristics ( I SD – V GS ) of the hyper-FET and the FinFET (stand-alone). ( c ) The p-hyper-FET shows a ∼ 60 % higher ON-state current ( I SD,ON ) in comparison to the stand-alone FinFET over a gate-voltage window of −0.5 V at matched OFF-state current. ( d ) Output characteristics ( I SD – V DS ) of the p-hyper-FET and the conventional FinFET. Full size image Figure 3a illustrates a scaled hyper-FET consisting of a scaled In 0.7 Ga 0.3 As quantum-well multi-channel FinFET ( L g =500 nm) (see Supplementary Fig. 4 and Supplementary Note 4 for fabrication method) in series with VO 2 ( =200 nm; =1 μm). Figure 3b shows the transfer characteristics of the hyper-FET (and the stand-alone FinFET) exhibiting a ‘gate controlled’ abrupt turn-ON/turn-OFF associated with the IMT/MIT in VO 2 , respectively. The direct comparison of the hyper-FET with the stand-alone FinFET reveals an improved I DS,ON / I DS,OFF ratio over a V GS range of 0.8 V, and thus a ∼ 20% enhancement in I DS,ON at matched I DS,OFF ( Fig. 3c ). The corresponding output characteristics of the hyper-FET and its constituent FinFET, shown in Fig. 3d , also reflect the I DS enhancement. We also demonstrate a p-type hyper-FET since complementary operation, similar to the complementary metal-oxide-semiconductor (CMOS) logic family, is imperative for low standby-power digital applications. Two-terminal VO 2 devices exhibit reversible switching in both positive and negative voltage polarities ( Supplementary Fig. 1 ) which allows for electrical integration with a p-channel FinFET to enable p-type hyper-FET operation. Figure 4a shows the schematic of a p-hyper-FET constructed using a p-channel Ge quantum-well multi-channel FinFET (see Supplementary Fig. 4 and Supplementary Note 4 for fabrication method) in series with VO 2 ( =200 nm; =1 μm). Figure 4b,d shows the transfer characteristics and the corresponding output characteristics of the p-hyper-FET and its constituent FinFET, respectively. The p-hyper-FET also exhibits an enhanced I SD,ON / I SD,OFF ratio over a V GS range of −0.5 V, and thus a ∼ 60% enhancement in I SD,ON at matched I SD,OFF ( Fig. 4c ). The hyper-FET is a device concept that harnesses the phase transition in the IMT material, VO 2 , to enable room temperature, steep-slope, n-type and p-type transistor operation with enhanced performance. These experimental results motivate the realization of a scaled, monolithic hyper-FET design entailing hetero-integration of the IMT material with the conventional FET [44] , [45] , [46] , [47] , [48] . Such an integrated device would have to include careful design considerations for minimizing the device ‘foot-print’ [44] , reducing potential self-heating effects as well as ensuring low-contact resistance of both the conventional MOSFET, which can adversely affect its ON-state current (and therefore that of the hyper-FET), and that of the VO 2 , which may possibly affect the magnitude of abrupt current change across the IMT. Further, scaling and optimizing the VO 2 and the MOSFET properties to enable a scaled hyper-FET device with low OFF-state leakage current relevant to low-power circuit applications [49] , and reduced hysteresis with a complete rail-to-rail swing in a complementary configuration (some of the design considerations are discussed in Supplementary Note 5 and Supplementary Fig. 5 ) will be key factors in realizing a hyper-FET-based hardware platform that can augment current state-of-the-art technology [49] . The hyper-FET, demonstrated here, is a manifestation of a design methodology that consolidates the unique properties of phase transition materials like abrupt and reversible resistivity switching, arising from collective carrier dynamics and usually inaccessible in a conventional semiconductor, with the robust field-induced switching dynamics of a conventional MOSFET. Our approach harnesses the abrupt IMT in VO 2 in the much-desired three-terminal transistor configuration, circumventing the need for direct electric field-induced phase transition. Furthermore, the generality of the hyper-FET design also facilitates this transistor architecture to be extended to other insulator–metal transition systems, [50] , [51] , [52] thus opening the doors to using electronic phase transition materials in digital applications. How to cite this article: Shukla, N. et al . A steep-slope transistor based on abrupt electronic phase transition. Nat. Commun. 6:7812 doi: 10.1038/ncomms8812 (2015).